The internal Cdc20 binding site in BubR1 facilitates both spindle assembly checkpoint signalling and silencing Improperly attached kinetochores activate the spindle assembly checkpoint (SAC) and by an unknown mechanism catalyse the binding of two checkpoint proteins, Mad2 and BubR1, to Cdc20 forming the mitotic checkpoint complex (MCC). Here, to address the functional role of Cdc20 kinetochore localization in the SAC, we delineate the molecular details of its interaction with kinetochores. We find that BubR1 recruits the bulk of Cdc20 to kinetochores through its internal Cdc20 binding domain (IC20BD). We show that preventing Cdc20 kinetochore localization by removal of the IC20BD has a limited effect on the SAC because the IC20BD is also required for efficient SAC silencing. Indeed, the IC20BD can disrupt the MCC providing a mechanism for its role in SAC silencing. We thus uncover an unexpected dual function of the second Cdc20 binding site in BubR1 in promoting both efficient SAC signalling and SAC silencing. Accurate chromosome segregation during mitosis is ensured by the spindle assembly checkpoint (SAC), which is a conserved mechanism requiring the Aurora B, Mad1, Mad2, Mps1, Bub1, BubR1 (Mad3 in yeast) and Bub3 proteins [1] , [2] . The proper attachment of microtubules to kinetochores is monitored by the SAC and a single incorrectly attached kinetochore is able to activate the checkpoint [3] , [4] . The SAC inhibits chromosome segregation and mitotic exit by blocking the degradation of Securin and Cyclin B1, respectively. Both of these proteins are targeted for degradation by an E3 ubiquitin ligase, the anaphase promoting complex/cyclosome (APC/C) in complex with its co-activator Cdc20 (ref. 5 ). APC/C activity is inhibited by the cooperative binding of three checkpoint proteins, Mad2, BubR1 and Bub3, to Cdc20, which results in the formation of the mitotic checkpoint complex (MCC) [6] , [7] , [8] , [9] , [10] , [11] . Mad2 can bind stably to Cdc20 independently of BubR1, while BubR1 requires Mad2 for its stable association with Cdc20 (refs 12 , 13 , 14 , 15 ). Bub3 does not directly bind to Cdc20 but is required for kinetochore recruitment of BubR1 (refs 16 , 17 , 18 ). Mad2 binds to a short conserved sequence in the N terminus of Cdc20 while BubR1 interacts with the WD40 domain of Cdc20 and additional contacts between Mad2 and BubR1 stabilize the entire MCC [19] , [20] . The protein p31 binds to Mad2 and removes it from the MCC leading to sub stoichiometric levels of Mad2 in the MCC [21] . An N-terminal KEN box motif in BubR1 is critical for stable binding to Cdc20 and binds to conserved residues on the top side of the WD40 domain [17] , [19] , [22] , [23] , [24] , [25] . BubR1 in vertebrates also contains an internal Cdc20 binding domain (referred to here as IC20BD) that binds the Cdc20 WD40 domain in a Mad2-independent manner [6] , [26] , [27] . IC20BD spans residues 490–560 in human BubR1 and binding to Cdc20 depends on a conserved stretch of six amino acids within this otherwise poorly conserved part of BubR1 (ref. 26 ). The exact function of the IC20BD is not clear, but it appears largely dispensable for SAC signalling [14] , [17] , [28] . Cdc20 inhibitory complexes might be assembled at the kinetochore as the removal of outer kinetochore proteins inactivates the checkpoint [29] . In line with this, a small fraction of all checkpoint proteins as well as Cdc20 accumulates at unattached kinetochores and turns over rapidly here [30] , [31] , [32] . Indeed, elegant biochemical experiments have shown that kinetochores can stimulate complex formation between Mad2 and Cdc20 (ref. 13 ). Understanding how the kinetochore stimulates the binding of checkpoint proteins to Cdc20 is a key unresolved question but requires a detailed understanding of how Cdc20 interacts with kinetochores, which is currently missing. Here, we show that the IC20BD of BubR1 is the major kinetochore receptor for Cdc20 and that this domain has dual functions during SAC—both in signalling and silencing. We propose that this dual function could couple BubR1 localization to MCC production or disassembly. Localization of Cdc20 to kinetochores requires BubR1 To understand the mechanism of Cdc20 kinetochore localization, we first aimed at identifying the kinetochore receptor during prometaphase. A Cdc20 monoclonal antibody stained kinetochores, and this staining was absent in cells depleted of Cdc20 by RNAi showing that it is specific ( Supplementary Fig. 1a ). Epitope mapping by peptide array identified an epitope in the N terminus of Cdc20 and the antibody could immunoprecipitate MCC components ( Supplementary Fig. 1b,c ). We analysed Cdc20 localization as HeLa cells progressed through an unperturbed mitosis and observed that the levels were highest in prometaphase at unattached kinetochores and decreased in metaphase and anaphase ( Supplementary Fig. 1d,e ). Thus, Cdc20 shows the same localization pattern as canonical SAC components as expected and argued that Cdc20 was very likely recruited to kinetochores through interactions with SAC components. To determine which protein(s) Cdc20 interacts with at the kinetochore, we focused on Mad2 and BubR1, as these were obvious candidates. We performed RNAi depletion of BubR1 and Mad2 ( Fig. 1a–c and Supplementary Fig. 1f for depletion efficiency). The depletion of BubR1 resulted in an ≈65% decrease in Cdc20 kinetochore levels, while Mad2 depletion resulted in an ≈35% increase ( Fig. 1b,c ). 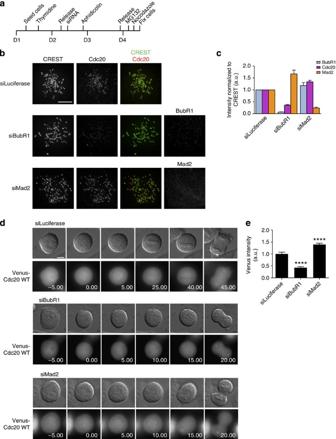Figure 1: Recruitment of Cdc20 to kinetochores requires BubR1. (a) Schematic of protocol used to synchronize cells and deplete specific proteins using RNAi. (b) Cells depleted of the indicated proteins were stained for CREST and Cdc20 and BubR1 or Mad2 to check for depletion efficiency. Scale bar, 5 μm. (c) Quantification of Cdc20, BubR1 and Mad2 kinetochore levels in cells treated with the indicated RNAi oligos. The fluorescence from the threez-stacks (200 nm apart) encompassing the bulk kinetochore fluorescent intensity was used and normalized to the CREST signal. Cells were co-stained for Mad2 or BubR1 to ensure that only cells with efficient depletion were analysed. At least 80 kinetochore pairs from eight cells were quantified and the mean and s.e.m. is indicated. (d) Stable HeLa cell line expressing Venus-Cdc20 was treated with the indicated RNAi oligos and the localization of Venus-Cdc20 followed by time-lapse microscopy. Scale bar, 10 μm. (e) Quantification of Venus-Cdc20 at kinetochores in the movies in (d). The signal was quantified from a singlez-section and in the frame right after NEBD. A total number of 50 kinetochores from 10 cells were analyzed for each condition and the mean and s.e.m. indicated. An unpairedt-test was performed for statistical analysis (****P<0.0001) and compared with the control-treated cells. Figure 1: Recruitment of Cdc20 to kinetochores requires BubR1. ( a ) Schematic of protocol used to synchronize cells and deplete specific proteins using RNAi. ( b ) Cells depleted of the indicated proteins were stained for CREST and Cdc20 and BubR1 or Mad2 to check for depletion efficiency. Scale bar, 5 μm. ( c ) Quantification of Cdc20, BubR1 and Mad2 kinetochore levels in cells treated with the indicated RNAi oligos. The fluorescence from the three z -stacks (200 nm apart) encompassing the bulk kinetochore fluorescent intensity was used and normalized to the CREST signal. Cells were co-stained for Mad2 or BubR1 to ensure that only cells with efficient depletion were analysed. At least 80 kinetochore pairs from eight cells were quantified and the mean and s.e.m. is indicated. ( d ) Stable HeLa cell line expressing Venus-Cdc20 was treated with the indicated RNAi oligos and the localization of Venus-Cdc20 followed by time-lapse microscopy. Scale bar, 10 μm. ( e ) Quantification of Venus-Cdc20 at kinetochores in the movies in ( d ). The signal was quantified from a single z -section and in the frame right after NEBD. A total number of 50 kinetochores from 10 cells were analyzed for each condition and the mean and s.e.m. indicated. An unpaired t -test was performed for statistical analysis (**** P <0.0001) and compared with the control-treated cells. Full size image We used a live cell approach to further investigate the role of Mad2 and BubR1 in Cdc20 kinetochore localization. To this end, we generated a stable HeLa cell line expressing Venus-Cdc20 (for expression levels see Supplementary Fig. 1g ), which has previously been shown to complement the Cdc20 RNAi phenotype [12] , [33] . This cell line and all other cell lines described here are stable isogenic inducible cell lines made using a HeLa FRT/TRex cell line. When cells expressing Venus-Cdc20 entered mitosis, Cdc20 accumulated on kinetochores and this signal decreased on alignment of chromosomes ( Fig. 1d , Supplementary Movie 1 ). In an unperturbed mitosis Cdc20 kinetochore localization depended on BubR1 but not on Mad2 ( Fig. 1d , Supplementary Movies 2 and 3 ). Quantification of the kinetochore intensity of Venus-Cdc20 from the movies revealed similar results as obtained with endogenous Cdc20 ( Fig. 1e ). For this analysis we only analysed cells that progressed rapidly through mitosis ensuring that the RNAi against BubR1 and Mad2 had worked (see also Supplementary Fig. 1h for phenotypic effect of Mad2 and BubR1 RNAi). Similar qualitative results were obtained in cells treated with nocodazole ( Supplementary Fig. 1i ). Our results reveal a role for BubR1 in the recruitment of Cdc20 to kinetochores, similar to that reported in mice and flies [27] , [34] . BubR1 appears to be a major receptor for Cdc20 at kinetochores, but additional receptor(s) likely exist as ≈35% Cdc20 remains after very efficient BubR1 depletion. In agreement with this, we have found that depletion of KNL1 results in a more efficient removal of Cdc20 from kinetochores, which is not due to more efficient BubR1 removal from kinetochores ( Supplementary Fig. 1i ). Given that BubR1 played a clear role in recruiting Cdc20 to kinetochores, we here focus our efforts on understanding the interaction between these two proteins at kinetochores. Cdc20 KEN box binding is needed for kinetochore localization The interaction between Cdc20 and BubR1 within the MCC strongly depends on binding of the N-terminal KEN box of BubR1 to residues of the WD40 domain of Cdc20 (refs 19 , 25 ). To determine whether this interaction was still required for kinetochore localization of Cdc20, we mutated amino acids 377–380 of Cdc20 to alanine (mutant referred to as Cdc20 4A), as the available Cdc20-BubR1 structures predict this should disrupt KEN-box binding of Cdc20 ( Fig. 2a ) [19] , [25] . 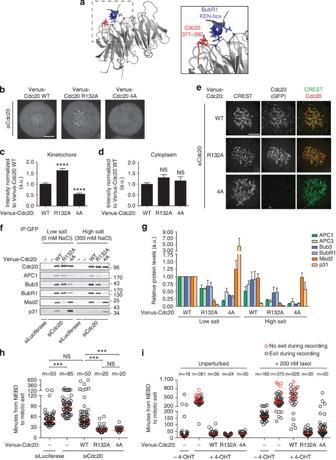Figure 2: A novel Cdc20 mutant specifically defective in BubR1 binding. (a) The structure of human Cdc20 bound to the BubR1 KEN-box motif (blue) (PDB: 4GGD) with the residues mutated in Cdc20 4A in red. (b) Stable HeLa cell lines expressing the indicated Cdc20 proteins were analysed by live cell spinning disc confocal microscopy and representative still images are shown. Scale bar, 10 μm. (c) Quantification of Cdc20 intensity at the kinetochores from the experiment shown in (b). A total of 50 kinetochores from 10 different cells were analysed for each condition. Cdc20 kinetochore signal was determined using the ImageJ software and mean and s.e.m. are shown. An unpairedt-test was used for statistical analysis. (****P<0.0001). (d) The Cdc20 intensity in the cytoplasm was measured from the images acquired with the spinning disc from the 10 cells used for the analysis in (c). An unpairedt-test was used for statistical analysis. (e) Stable HeLa cell lines expressing the indicated Cdc20 proteins were arrested by nocodazole and MG132, and stained for CREST and Cdc20 using a GFP specific antibody. Scale bar, 5 μm. (f) Stable HeLa cell lines expressing the indicated Cdc20 proteins were arrested in nocodazole and MG132 and cells collected by mitotic shake-off. Venus-Cdc20 proteins were purified using a GFP affinity resin and washed with either a low salt buffer or high salt buffer as indicated. The composition of proteins associated with Cdc20 was determined by blotting for the indicated proteins. (g) Quantification of the proteins bound to Venus-Cdc20 proteins was determined. The mean and s.e.m. of two independent experiments are shown. (h) Stable HeLa cells were treated with a control RNAi oligo (Luciferase) or depleted of Cdc20 and then complemented with the different Venus-Cdc20 proteins as indicated. Each circle represents a single cell analysed (at least 60 cells were analysed for each condition) and the red line indicates the median (m). A Mann–Whitney test was performed for statistical analysis. (i) Mouse embryonic fibroblasts (MEFs) were depleted of Cdc20 by addition of 4-OHT 24 h before imaging and complemented with the indicated Venus-Cdc20 proteins. At least 25 cells were analysed per condition and a Mann–Whitney test was used for statistical analysis. Median time (m) is indicated for each condition. Figure 2: A novel Cdc20 mutant specifically defective in BubR1 binding. ( a ) The structure of human Cdc20 bound to the BubR1 KEN-box motif (blue) (PDB: 4GGD) with the residues mutated in Cdc20 4A in red. ( b ) Stable HeLa cell lines expressing the indicated Cdc20 proteins were analysed by live cell spinning disc confocal microscopy and representative still images are shown. Scale bar, 10 μm. ( c ) Quantification of Cdc20 intensity at the kinetochores from the experiment shown in ( b ). A total of 50 kinetochores from 10 different cells were analysed for each condition. Cdc20 kinetochore signal was determined using the ImageJ software and mean and s.e.m. are shown. An unpaired t -test was used for statistical analysis. (**** P <0.0001). ( d ) The Cdc20 intensity in the cytoplasm was measured from the images acquired with the spinning disc from the 10 cells used for the analysis in ( c ). An unpaired t -test was used for statistical analysis. ( e ) Stable HeLa cell lines expressing the indicated Cdc20 proteins were arrested by nocodazole and MG132, and stained for CREST and Cdc20 using a GFP specific antibody. Scale bar, 5 μm. ( f ) Stable HeLa cell lines expressing the indicated Cdc20 proteins were arrested in nocodazole and MG132 and cells collected by mitotic shake-off. Venus-Cdc20 proteins were purified using a GFP affinity resin and washed with either a low salt buffer or high salt buffer as indicated. The composition of proteins associated with Cdc20 was determined by blotting for the indicated proteins. ( g ) Quantification of the proteins bound to Venus-Cdc20 proteins was determined. The mean and s.e.m. of two independent experiments are shown. ( h ) Stable HeLa cells were treated with a control RNAi oligo (Luciferase) or depleted of Cdc20 and then complemented with the different Venus-Cdc20 proteins as indicated. Each circle represents a single cell analysed (at least 60 cells were analysed for each condition) and the red line indicates the median (m). A Mann–Whitney test was performed for statistical analysis. ( i ) Mouse embryonic fibroblasts (MEFs) were depleted of Cdc20 by addition of 4-OHT 24 h before imaging and complemented with the indicated Venus-Cdc20 proteins. At least 25 cells were analysed per condition and a Mann–Whitney test was used for statistical analysis. Median time (m) is indicated for each condition. Full size image We imaged live cells expressing Venus-Cdc20 4A by spinning disc confocal microscopy and observed weaker kinetochore localization of Cdc20 4A compared with wild-type Cdc20 ( Fig. 2b,c ). In contrast, when we mutated the Mad2 binding site of Cdc20 by introducing the R132A mutation, there was an increase in Cdc20 kinetochore levels ( Fig. 2b,c ). These differences were not due to differences in the overall expression levels of the different Cdc20 proteins ( Fig. 2d ). The kinetochore localization pattern of the Cdc20 mutants was also confirmed by staining the stable cell lines for exogenous Cdc20 ( Fig. 2e ), and this is in agreement with the results from our RNAi depletion of Mad2 and BubR1 ( Fig. 1 ). To ensure that the Cdc20 4A was indeed a functional protein and its inability to locate to kinetochores was not due to misfolding, we further analysed this mutant. First, we determined the ability of Cdc20 4A to co-immunoprecipitate known interactors from mitotic cells when endogenous Cdc20 was depleted ( Fig. 2f,g ). Cdc20 4A showed a clear reduction in BubR1-Bub3 binding but maintained binding to Mad2 as predicted. In agreement with the fission yeast MCC structure [19] , which revealed that BubR1 and p31 compete for the same binding site on Mad2, more p31 comet co-purified with Cdc20 4A. Indeed, Mad2 dissociated much more readily from Cdc20 4A when the SAC was silenced ( Supplementary Fig. 2a ). As predicted, the Cdc20 R132A mutant had reduced Mad2 binding but still maintained some binding to BubR1-Bub3, although at reduced levels. We next analysed mitotic progression in stable HeLa cells expressing Venus-tagged Cdc20, Cdc20 R132A and Cdc20 4A that were depleted of endogenous Cdc20. The depletion of Cdc20 delayed cells in mitosis and this could be rescued by expressing Venus-Cdc20 ( Fig. 2h ). The expression of Cdc20 R132A and Cdc20 4A allowed mitotic progression supporting that the mutant proteins were functional and properly folded and this was further confirmed by in vitro APC/C ubiquitination assays ( Supplementary Fig. 2b ). Furthermore, both Cdc20 R132A and Cdc20 4A progressed faster through mitosis ( Fig. 2h ) in agreement with the biochemical analysis showing weaker binding to MCC components. As the depletion of Cdc20 by RNAi in HeLa cells does not give a robust mitotic arrest, we also analysed the ability of Cdc20 4A to support mitotic progression in mouse embryonic fibroblasts (MEFs). We obtained MEFs from the Malumbres lab where exon 2 of Cdc20 is flanked by loxP sites and can be efficiently removed by Cre recombinase [35] . The MEFs were transfected with the different Venus-Cdc20 constructs (human and mouse Cdc20 are almost identical), and removal of endogenous Cdc20 was induced by addition of 4-hydroxytamoxifen (4-OHT) 24 h before time-lapse imaging. Without the introduction of exogenous Cdc20 there was a strong mitotic delay indicative of efficient Cdc20 removal ( Fig. 2i , Supplementary Fig. 2c ). This was fully suppressed by reintroducing the different forms of Cdc20, showing that Cdc20 4A and Cdc20 R132A are functional ( Fig. 2i , Supplementary Fig. 2c ). When we challenged the MEFs with taxol to activate the SAC, a prolonged mitotic arrest was observed when we reintroduced Cdc20 but not Cdc20 R132A and Cdc20 4A confirming that these mutants are checkpoint defective ( Fig. 2i ). The analysis of Cdc20 4A reveals that this is a functional protein able to interact with Mad2 but defective in stable binding to BubR1-Bub3 and therefore unable to support SAC signalling. The failure of Cdc20 4A to efficiently locate to kinetochores further supports the role of BubR1 as a kinetochore receptor for Cdc20. The IC20BD of BubR1 recruits Cdc20 to kinetochores As Cdc20 4A is inefficiently recruited to kinetochores it suggested to us that the N-terminal KEN box of BubR1 recruits Cdc20 to kinetochores. To test this we generated a panel of stable cell lines expressing inducible Venus-tagged siRNA-resistant BubR1 constructs ( Fig. 3a ). We then depleted endogenous BubR1 and induced the expression of exogenous BubR1 and treated cells with nocodazole before fixation and staining. We stained with a BubR1 antibody recognizing an epitope present in all the BubR1 constructs assayed and only analysed cells that had a similar level of BubR1 at kinetochores as control-treated cells. The kinetochore localization of Cdc20 could be restored to normal levels by expressing exogenous BubR1 ( Fig. 3b–e ). Surprisingly, a BubR1 mutant in which the first KEN box was mutated to AAA (BubR1 KEN/AAA) also efficiently recruited Cdc20 to kinetochores ( Fig. 3b–e ). BubR1 KEN/AAA was clearly defective in forming the MCC as predicted (see Fig. 4d ). When we compared the ability of BubR1 1–483 and BubR1 1–715 in recruiting Cdc20 to kinetochores there was a striking difference. BubR1 1–715 clearly recruited Cdc20, while BubR1 1–483 did not ( Fig. 3b–e ). The major difference between these two BubR1 constructs is that BubR1 1–715 contains the IC20BD. In agreement with this, when we deleted the IC20BD of BubR1 (BubR1 Δ490–560), the BubR1-dependent kinetochore localization of Cdc20 was lost ( Fig. 3b–e ) indicating that the IC20BD and not the N-terminal KEN box of BubR1 recruits Cdc20 to the kinetochores. Removal of six conserved residues of the IC20BD (BubR1 Δ530–535) was enough to prevent Cdc20 kinetochore localization. Both BubR1 Δ490–560 and BubR1 Δ530–35 appeared to be folded properly as they migrated as wild-type BubR1 on a size exclusion column with no signs of larger aggregates ( Supplementary Fig. 3a ). Indeed a short peptide encompassing this region of BubR1, but not a mutant peptide, could bind purified Cdc20 arguing that the loss of Cdc20 kinetochore localization on deletion of the IC20BD is due to loss of a Cdc20 binding site and not misfolding of BubR1 ( Supplementary Fig. 3b ). In agreement with this a fragment of BubR1 encompassing the IC20BD could recruit Cdc20 to kinetochores ( Supplementary Fig. 3c ). On overexpression (~300-fold endogenous levels) of Venus-tagged BubR1 proteins encompassing the IC20BD in HEK293 cells, we could detect Cdc20 binding confirming previous observations ( Supplementary Fig. 3d,e ) [26] , [27] . However, at endogenous levels, IC20BD-containing BubR1 fragments do not co-purify detectable levels of Cdc20 (data not shown). This could either be due to a weak interaction that is not maintained during our purification conditions or that only a small fraction of BubR1 is interacting with Cdc20 through its IC20BD. 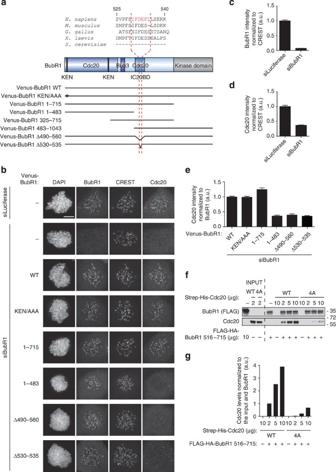Figure 3: The internal Cdc20 binding site of BubR1 recruits Cdc20 to kinetochores. (a) Schematic of human BubR1 and the location of Cdc20 binding sites and Bub3 binding site as well as the pseudo-kinase domain. Alignment of the region encompassing residues 530–535 of human BubR1 is shown on top and the different constructs used are indicated below. The BubR1 KEN/AAA has the first KEN-box mutated to AAA. (b) Stable HeLa cell lines expressing the different Venus-BubR1 siRNA resistant constructs were used to determine the domains in BubR1 required for Cdc20 kinetochore localization. In brief, cells were treated with a control RNAi oligo (Luciferase) or a BubR1 RNAi oligo and then arrested in mitosis using nocodazole treatment and the proteasome inhibitor, MG132. BubR1 RNAi-treated cells were complemented with the indicated Venus-BubR1 constructs. Cells were stained for BubR1, CREST and Cdc20. Scale bar, 5 μm (c,d). The kinetochore levels of BubR1 (c) and Cdc20 (d) normalized to CREST in control and BubR1-depleted cells. At least 80 kinetochore pairs from eight different cells were analysed, and the mean and s.e.m. are indicated. (e) The level of Cdc20 at kinetochores in cells complemented with the indicated Venus-BubR1 constructs was determined. Only cells with endogenous levels of BubR1 at kinetochores were used for this analysis. At least 80 kinetochore pairs from eight different cells were analysed, and the mean and s.e.m. are indicated. (f) Binding of Cdc20 and Cdc20 4A to BubR1 516–715 was determined by binding 10 μg recombinant FLAG-HA-BubR1 516–715 to FLAG affinity beads and incubating these with increasing concentrations of Strep-His tagged Cdc20 or Cdc20 4A expressed and purified from HEK293 cells. The beads were washed and bound proteins were eluted and analysed by western blot. (g) Quantification of western blot in (f) using Licor technology. Experiment in (f,g) is representative of two independent experiments. Figure 3: The internal Cdc20 binding site of BubR1 recruits Cdc20 to kinetochores. ( a ) Schematic of human BubR1 and the location of Cdc20 binding sites and Bub3 binding site as well as the pseudo-kinase domain. Alignment of the region encompassing residues 530–535 of human BubR1 is shown on top and the different constructs used are indicated below. The BubR1 KEN/AAA has the first KEN-box mutated to AAA. ( b ) Stable HeLa cell lines expressing the different Venus-BubR1 siRNA resistant constructs were used to determine the domains in BubR1 required for Cdc20 kinetochore localization. In brief, cells were treated with a control RNAi oligo (Luciferase) or a BubR1 RNAi oligo and then arrested in mitosis using nocodazole treatment and the proteasome inhibitor, MG132. BubR1 RNAi-treated cells were complemented with the indicated Venus-BubR1 constructs. Cells were stained for BubR1, CREST and Cdc20. Scale bar, 5 μm ( c , d ). The kinetochore levels of BubR1 ( c ) and Cdc20 ( d ) normalized to CREST in control and BubR1-depleted cells. At least 80 kinetochore pairs from eight different cells were analysed, and the mean and s.e.m. are indicated. ( e ) The level of Cdc20 at kinetochores in cells complemented with the indicated Venus-BubR1 constructs was determined. Only cells with endogenous levels of BubR1 at kinetochores were used for this analysis. At least 80 kinetochore pairs from eight different cells were analysed, and the mean and s.e.m. are indicated. ( f ) Binding of Cdc20 and Cdc20 4A to BubR1 516–715 was determined by binding 10 μg recombinant FLAG-HA-BubR1 516–715 to FLAG affinity beads and incubating these with increasing concentrations of Strep-His tagged Cdc20 or Cdc20 4A expressed and purified from HEK293 cells. The beads were washed and bound proteins were eluted and analysed by western blot. ( g ) Quantification of western blot in ( f ) using Licor technology. Experiment in ( f , g ) is representative of two independent experiments. 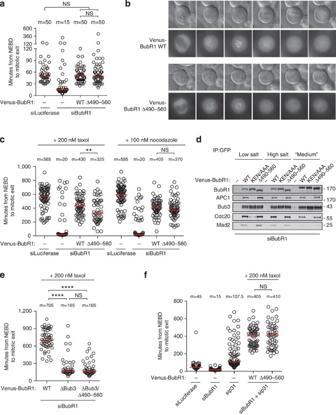Figure 4: The internal Cdc20 binding site of BubR1 contributes to SAC signalling during a taxol-induced arrest. (a) Mitotic progression in HeLa cells stably expressing similar levels of Venus-BubR1 or Venus-BubR1 Δ490–560 and depleted of endogenous BubR1 was determined by time-lapse microscopy. This was compared with Luciferase RNAi and BubR1 RNAi-treated cells. Each circle represents a single cell analysed (at least 50 cells were analyzed per condition) and the red line indicates the median (m). A Mann–Whitney test was used for statistical analysis. (b) Still images from the time-lapse movies of Venus-BubR1 and Venus-BubR1 Δ490–560. Scale bar, 10 μm. (c) Similar to (a) but cells was challenged with either 200 nM taxol or 100 nM nocodazole as indicated. The red line indicates the median (m) and each circle represents a single cell analysed (at least 50 cells were analysed per condition). A Mann–Whitney test was used for statistical analysis. (d) The indicated Venus-BubR1 proteins were purified from taxol-arrested cells using a GFP affinity resin and washed with different salt conditions, as indicated. The binding to the indicated proteins was analysed by western blotting. (e) HeLa cells stably expressing similar levels of Venus-BubR1, Venus-BubR1 ΔBub3 or Venus-BubR1 ΔBub3/Δ490–560 and depleted of endogenous BubR1 were treated with 200 nM taxol and their mitotic progression was followed by time-lapse microscopy. Each circle represents a single cell analysed (at least 40 cells were analysed per condition) and the red bars indicate the medians (m). A Mann–Whitney test was used for statistical analysis. (f) HeLa cells were depleted of BubR1 and/or p31cometas indicated. Luciferase knockdown was included as control. BubR1 depletion was complemented with Venus-BubR1 or Venus-BubR1 Δ490–560 as indicated and 200 nM taxol was added before filming. Each circle represents a single cell analysed and at least 50 cells were analysed per condition. Medians (m) are shown in red and a Mann–Whitney test was used for the statistical analysis. Full size image Figure 4: The internal Cdc20 binding site of BubR1 contributes to SAC signalling during a taxol-induced arrest. ( a ) Mitotic progression in HeLa cells stably expressing similar levels of Venus-BubR1 or Venus-BubR1 Δ490–560 and depleted of endogenous BubR1 was determined by time-lapse microscopy. This was compared with Luciferase RNAi and BubR1 RNAi-treated cells. Each circle represents a single cell analysed (at least 50 cells were analyzed per condition) and the red line indicates the median (m). A Mann–Whitney test was used for statistical analysis. ( b ) Still images from the time-lapse movies of Venus-BubR1 and Venus-BubR1 Δ490–560. Scale bar, 10 μm. ( c ) Similar to ( a ) but cells was challenged with either 200 nM taxol or 100 nM nocodazole as indicated. The red line indicates the median (m) and each circle represents a single cell analysed (at least 50 cells were analysed per condition). A Mann–Whitney test was used for statistical analysis. ( d ) The indicated Venus-BubR1 proteins were purified from taxol-arrested cells using a GFP affinity resin and washed with different salt conditions, as indicated. The binding to the indicated proteins was analysed by western blotting. ( e ) HeLa cells stably expressing similar levels of Venus-BubR1, Venus-BubR1 ΔBub3 or Venus-BubR1 ΔBub3/Δ490–560 and depleted of endogenous BubR1 were treated with 200 nM taxol and their mitotic progression was followed by time-lapse microscopy. Each circle represents a single cell analysed (at least 40 cells were analysed per condition) and the red bars indicate the medians (m). A Mann–Whitney test was used for statistical analysis. ( f ) HeLa cells were depleted of BubR1 and/or p31 comet as indicated. Luciferase knockdown was included as control. BubR1 depletion was complemented with Venus-BubR1 or Venus-BubR1 Δ490–560 as indicated and 200 nM taxol was added before filming. Each circle represents a single cell analysed and at least 50 cells were analysed per condition. Medians (m) are shown in red and a Mann–Whitney test was used for the statistical analysis. Full size image KEN-box binding residues of Cdc20 binds the IC20BD Initially, we had hypothesized that the defect in kinetochore localization of Cdc20 4A was due to its inability to bind the N-terminal KEN box of BubR1. However, given our observation that BubR1 KEN/AAA still recruited Cdc20 to kinetochores this result was inconsistent with this model. We reasoned that possibly the same residues of Cdc20 binding to the N-terminal KEN-box of BubR1 are also required for binding to IC20BD, even though the IC20BD does not contain a KEN-box motif. To test this hypothesis, we expressed Cdc20 and Cdc20 4A in HEK293 cells and purified the proteins using a strep-tag. We then compared the ability of the Cdc20 proteins to bind a recombinant FLAG-tagged fragment of BubR1 (amino acids 516–715) that encompasses the conserved residues of the IC20BD that we found necessary for Cdc20 kinetochore recruitment. The BubR1 fragment was first bound to beads using its FLAG tag, next purified Cdc20 and Cdc20 4A were titrated in and following incubation, the beads were washed. Proteins bound to the beads were analysed by both quantitative western blotting and by Coomassie staining ( Fig. 3f,g and Supplementary Fig. 3f ). From these experiments, it was clear that Cdc20 bound BubR1 516–715 while this binding was strongly reduced in Cdc20 4A explaining its reduced kinetochore localization. Cdc20 kinetochore localization facilitates SAC signalling As the IC20BD of BubR1 was required for kinetochore localization of Cdc20, we anticipated that it could contribute to SAC signalling, although previous work has shown that the N-terminal half of BubR1 is largely sufficient for a functional SAC [14] , [17] , [27] . To analyse the function of IC20BD, we compared mitotic progression in stable cell lines depleted of endogenous BubR1 and complemented with either Venus-BubR1 or Venus-BubR1 Δ490–560 at close to endogenous levels ( Fig. 4a,b , Supplementary Fig. 4a ). We only analysed cells with comparable levels of BubR1 as judged from the intensity of the Venus signal. In an unperturbed mitosis, we did not observe any effect on mitotic progression when we removed residues 490–560 ( Fig. 4a,b ). We then challenged the cells with either taxol or nocodazole and monitored the length of mitotic arrest ( Fig. 4c ). In agreement with previous reports, taxol-arrested cells had very few or no Mad2-positive kinetochores, while all kinetochores in nocodazole-arrested cells were Mad2 positive ( Supplementary Fig. 4b ). In nocodazole-arrested cells, the median time of arrest was only slightly reduced in BubR1 Δ490–560 complemented cells (BubR1 t =405 min, BubR1 Δ490–560 t =370 min) but this was not statistically significant. In taxol-arrested cells, the length of mitotic arrest was significantly lower in BubR1 Δ490–560 (BubR1 t =430 min, BubR1 Δ490–560 t =325 min, P ≤0.01) but MCC formation was not detectably affected, likely reflecting that the biochemical assay is less sensitive in detecting small differences in MCC composition ( Fig. 4d ). A similar result was obtained with BubR1 Δ530–535 in taxol ( Supplementary Fig. 4c ). As the effect that we saw could be due either to the impaired binding of Cdc20 to the IC20BD of BubR1 or to Cdc20 impaired localization to the kinetochore, we prevented BubR1 kinetochore localization by mutating the Bub3 binding site in BubR1 (BubR1 E412K/E413K) and BubR1 Δ490–560 (referred to as BubR1 ΔBub3 and BubR1 ΔBub3/Δ490–560), which strongly reduced SAC strength ( Fig. 4e ). In this situation, we exclude the effect of BubR1 kinetochore localization and thereby also of Cdc20, so we can assess the importance of Cdc20 binding alone. The duration of a taxol-induced mitotic arrest was the same in BubR1 ΔBub3 and BubR1 ΔBub3/Δ490–560 complemented cells suggesting that it is not the binding of Cdc20 to IC20BD but the kinetochore localization of Cdc20 that contributes to SAC signalling in taxol ( Fig. 4e ). Our results therefore suggest that Cdc20 kinetochore localization by the IC20BD contributes to SAC signalling under conditions where Mad2 kinetochore levels are low likely by facilitating Mad2–Cdc20 complex formation. In agreement with this hypothesis, depletion of p31 comet , which stabilizes the Mad2-Cdc20 complex, resulted in similar timing of BubR1 and BubR1 Δ490–560 in taxol-treated cells ( Fig. 4f ). The IC20BD is required for SAC silencing Our analysis of the IC20BD reveals that it makes a small contribution to SAC signalling, despite being critical for Cdc20 kinetochore localization. This was puzzling as BubR1 kinetochore localization was critical for an efficient SAC ( Fig. 4e and ref. 17 ). However, we observed that in an unperturbed mitosis BubR1 ΔBub3/Δ490–560 complemented cells spent longer time in mitosis than BubR1 ΔBub3 (BubR1 ΔBub3/Δ490–560 t =67.5 min, BubR1 ΔBub3 t =50 min, Mann–Whitney test P ≤0.0001) ( Fig. 5a ). Thus, under conditions where the SAC is weakened and MCC production lowered, the IC20BD seemed important for cells to exit mitosis and thus had the opposite effect than observed in the taxol and nocodazole challenge experiments. This pointed to a role of the IC20BD in SAC silencing. 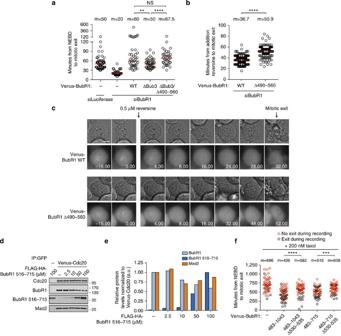Figure 5: The IC20BD is required for SAC silencing. (a) Stable HeLa cells were depleted of endogenous BubR1 or treated with control RNAi oligo (Luciferase). BubR1 knockdown was complemented by expression of Venus-BubR1, Venus-BubR1 ΔBub3 or Venus-BubR1 ΔBub3/Δ490–560 as indicated and mitotic progression was followed by time-lapse microscopy. Each circle represents a single cell analysed (at least 40 cells were analysed for each condition) and the median (m) is shown as a red bar. Statistical analysis was performed using a Mann–Whitney test. (b) Stable HeLa cell lines were depleted of endogenous BubR1 and complemented by expression of Venus-BubR1 or Venus-BubR1 Δ490–560 as indicated. Cells were arrested in mitosis with 100 nM nocodazole before filming and subsequently treated with 0.5 μM reversine to silence the SAC. Each circle represents a single cell analysed and at least 120 cells were analysed per condition. Red bars indicate means (m) and at-test was used for statistical analysis. (c) Representative still images from (b). Scale bar, 10 μm. (d,e) Venus-Cdc20 was purified from a stable HeLa cell line arrested in mitosis with nocodazole. The beads were incubated with increasing concentrations of recombinant FLAG-HA-BubR1 516–715 at room temperature for 1 h and afterwards washed. The binding of endogenous BubR1 and Mad2 to Venus-Cdc20 was analysed by western blot analysis and quantified using Licor technology. Representative of two independent experiments. (f) HeLa cells were transfected with the indicated BubR1 constructs and before filming 200 nM taxol was added. The time from NEBD to mitotic exit was measured by analysing the time-lapse movies and at least 50 cells were analysed per condition. Medians (m) are shown as red bars and a Mann–Whitney test was used for statistical analysis. Figure 5: The IC20BD is required for SAC silencing. ( a ) Stable HeLa cells were depleted of endogenous BubR1 or treated with control RNAi oligo (Luciferase). BubR1 knockdown was complemented by expression of Venus-BubR1, Venus-BubR1 ΔBub3 or Venus-BubR1 ΔBub3/Δ490–560 as indicated and mitotic progression was followed by time-lapse microscopy. Each circle represents a single cell analysed (at least 40 cells were analysed for each condition) and the median (m) is shown as a red bar. Statistical analysis was performed using a Mann–Whitney test. ( b ) Stable HeLa cell lines were depleted of endogenous BubR1 and complemented by expression of Venus-BubR1 or Venus-BubR1 Δ490–560 as indicated. Cells were arrested in mitosis with 100 nM nocodazole before filming and subsequently treated with 0.5 μM reversine to silence the SAC. Each circle represents a single cell analysed and at least 120 cells were analysed per condition. Red bars indicate means (m) and a t -test was used for statistical analysis. ( c ) Representative still images from ( b ). Scale bar, 10 μm. ( d , e ) Venus-Cdc20 was purified from a stable HeLa cell line arrested in mitosis with nocodazole. The beads were incubated with increasing concentrations of recombinant FLAG-HA-BubR1 516–715 at room temperature for 1 h and afterwards washed. The binding of endogenous BubR1 and Mad2 to Venus-Cdc20 was analysed by western blot analysis and quantified using Licor technology. Representative of two independent experiments. ( f ) HeLa cells were transfected with the indicated BubR1 constructs and before filming 200 nM taxol was added. The time from NEBD to mitotic exit was measured by analysing the time-lapse movies and at least 50 cells were analysed per condition. Medians (m) are shown as red bars and a Mann–Whitney test was used for statistical analysis. Full size image To directly test this, we challenged BubR1 and BubR1 Δ490–560 complemented cells with nocodazole and then treated them with reversine to silence the SAC and monitored time of exit by live cell microscopy ( Fig. 5b,c ). This revealed a clear role for the IC20BD in mediating efficient exit in that BubR1 exited with a median time of 36.7 min while BubR1 Δ490–560 took 50.9 min. Given that both the BubR1 N terminus and the IC20BD required the KEN box binding residues of Cdc20 for interaction, a possibility was that the IC20BD could facilitate SAC silencing through competition. To test this, we asked whether recombinant BubR1 516–715 could dissociate BubR1 from the MCC. Using a GFP affinity resin, we purified Venus-Cdc20 from nocodazole-arrested cells, which co-purified Mad2 and BubR1 ( Fig. 5d ). As previously discussed for Venus-BubR1, at close to endogenous levels of proteins we could not detect binding to the IC20BD, arguing that what we purify with Venus-Cdc20 is a mix of checkpoint complexes (Mad2-Cdc20-BubR1-Bub3, Cdc20-BubR1-Bub3 and Mad2-Cdc20). Next, we added increasing concentrations of recombinant BubR1 516–715 to our affinity purified Venus-Cdc20. Following a 1–h incubation at room temperature, the beads were washed and the amount of MCC components remaining bound to Cdc20 analysed by quantitative western blotting ( Fig. 5d,e ). With increasing concentrations of BubR1 516–715, we observed a gradual reduction of endogenous BubR1 bound to Cdc20 while the Mad2 levels were only slightly affected. In agreement with this when we overexpressed BubR1 fragments containing the IC20BD, but lacking their Bub3 binding site, the SAC was weakened in taxol-arrested cells. Importantly effective weakening of the SAC depended on the conserved residues of the IC20BD ( Fig. 5f ). Our results show that the IC20BD of BubR1 is required for efficient SAC silencing and a possible mechanism is by competing with the Mad3 homology region of BubR1 for binding to Cdc20. Here, we have dissected the major mechanism of Cdc20 kinetochore recruitment and show that this requires the IC20BD of BubR1 and KEN box binding residues of Cdc20. Preventing Cdc20 kinetochore localization by removing the IC20BD has a limited effect on the SAC but as the IC20BD is also required for SAC silencing these activities of the IC20BD are antagonizing each other potentially to make the checkpoint dynamic and responsive to BubR1 localization. Our finding that BubR1 is the major kinetochore receptor for Cdc20 in human cells, and that this in turn requires the internal Cdc20 binding site of BubR1, is in agreement with a number of previous observations. First, a clear role for BubR1 but not Mad2 in recruiting Cdc20 to kinetochores has been observed in flies and in mice [27] , [34] and fits with the temporal order of recruitment of BubR1 and Cdc20 (ref. 36 ). Second, removal of the Mad2 binding site from Cdc20 does not prevent its kinetochore localization in PtK 2 and LLC-PK1 cells similar to what we observe in human cells with Cdc20 R132A [30] , [31] . As the binding between Cdc20 and IC20BD does not require Mad2 binding to Cdc20 (refs 6 , 26 ), our data explain why Mad2 is not needed for bulk Cdc20 recruitment. Elegant FRAP studies of Cdc20 in PtK 2 cells revealed two equal sized populations of Cdc20 at kinetochores, one with a fast turnover and one with a slower turnover [30] . The Cdc20 population with a slower turnover was dependent on the N terminus of Cdc20 and an active SAC. The same study also detected two populations of BubR1 with similar slow and fast turnover as Cdc20. These data together with the data presented here suggests that Cdc20 is binding the IC20BD of both a slow and a fast pool of BubR1 at kinetochores and that the slow BubR1 pool depends on an active SAC ( Fig. 6 ). In flies there appears to be only a fast pool of Cdc20, which might reflect a difference in how BubR1 interacts with kinetochores [34] , [37] . 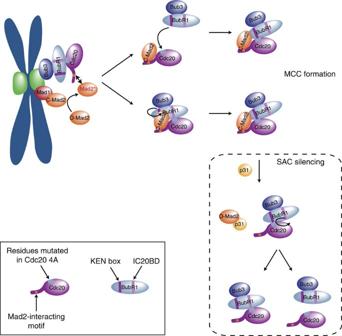Figure 6: Dual role of the IC20BD in regulating the SAC. At the kinetochore the IC20BD recruits Cdc20 to facilitate its interaction with Mad2 and potentially the formation of a partly assembled MCC. In the cytoplasm the IC20BD contributes to SAC silencing likely by competing for binding to Cdc20 with the N-terminal Mad3 homology region of BubR1. These two opposing activities of the IC20BD could make the SAC more dynamic and also couples MCC production or disassembly to BubR1 localization. Figure 6: Dual role of the IC20BD in regulating the SAC. At the kinetochore the IC20BD recruits Cdc20 to facilitate its interaction with Mad2 and potentially the formation of a partly assembled MCC. In the cytoplasm the IC20BD contributes to SAC silencing likely by competing for binding to Cdc20 with the N-terminal Mad3 homology region of BubR1. These two opposing activities of the IC20BD could make the SAC more dynamic and also couples MCC production or disassembly to BubR1 localization. Full size image Collectively, our data do not support that Cdc20 exists in MCC-like complexes at kinetochores as both preventing Mad2 binding or mutating the N-terminal KEN box of BubR1 did not affect Cdc20 localization. This suggests that the full assembly of the MCC occurs in the cytoplasm either through maturation of a partly assembled MCC or binding of soluble BubR1 to Mad2-Cdc20 ( Fig. 6 ). Although we find that BubR1 recruits the bulk of Cdc20 to kinetochores, our work also suggests that at least one other binding partner must exist at kinetochores as even after efficient BubR1 depletion ≈35% Cdc20 remains. The stronger effect of KNL1 RNAi could point to a role of Bub1 as an additional binding partner for Cdc20 at kinetochores and indeed human Bub1 has been shown to bind Cdc20 (ref. 38 ). Further experiments are needed to address the role of Bub1 in BubR1 and Cdc20 kinetochore localization. The exact function of the IC20BD of BubR1 has not been clear, and several studies have shown that it is not required for a functional SAC [14] , [17] . In the study from the Cleveland lab it was however noted that cells complemented with full-length BubR1 maintained a nocodazole induced arrest for longer time than cells complemented with BubR1 1–477 potentially revealing a role of the C-terminal half of BubR1 in prolonged arrest [14] . Although the IC20BD can inhibit Cdc20 activity in vitro [6] , our work and that of others indicate that in vivo the interaction of Cdc20 with this region of BubR1 is of either low affinity or restricted to binding a small proportion of Cdc20. Our comparison of BubR1 and BubR1 deleted of its IC20BD only revealed a small contribution of this domain to SAC signalling specifically in taxol-arrested cells. We favour that the function of the IC20BD is to weakly bind and hereby concentrate Cdc20 at kinetochores bringing it in proximity of the Mad1–Mad2 complex to facilitate Mad2–Cdc20 complex formation. The reason we favour this is that we only see a SAC defect when Mad2 signalling from kinetochores is low and this defect is suppressed by p31 comet removal. Furthermore the defect must relate to Cdc20 kinetochore localization as preventing BubR1 kinetochore localization abolishes the effect of removing the IC20BD. However, we cannot exclude that the IC20BD plays a more active role in the SAC. We also find a requirement of the IC20BD in SAC silencing and the true effect on the SAC on removal of the IC20BD is likely masked by this function. We roughly estimate the median times to be 50 min for BubR1 and 30 min for BubR1 Δ490–560 in an unperturbed mitosis without the effect of the IC20BD on SAC silencing. This is as severe an effect on the SAC as mutating the Bub3 binding site in BubR1. Our data would support a model in which the IC20BD contributes to SAC signalling by recruiting Cdc20 to kinetochores to facilitate interaction with Mad2 and in SAC silencing by destabilizing the BubR1–Cdc20 interaction within the MCC through competition ( Fig. 6 ). As these two activities of the IC20BD are counteracting each other, it depends on the experimental conditions what activity is the most dominant. This would explain why we only see a clear effect on the SAC in taxol-arrested cells where the role of the IC20BD in recruiting Cdc20 to kinetochores becomes very critical. BubR1 is recruited to improperly attached kinetochores and thus its function in recruiting Cdc20 to the kinetochore to facilitate interaction with Mad2 and at the same time recruiting PP2A [39] , [40] , [41] to stabilize kinetochore–microtubule interactions shows the remarkable ability of BubR1 to integrate important kinetochore activities through short interaction motifs. Once proper kinetochore–microtubule interactions are established, BubR1 leaves the kinetochore and the IC20BD then acts to destabilize the MCC for efficient mitotic exit. The dual function of the IC20BD thus elegantly couples SAC signalling or silencing to the localization of BubR1. Cloning and stable cell lines All constructs were cloned into pcDNA5/FRT/TO FLAG Venus (N-terminal tagging). Cdc20 and BubR1 and fragments thereof were amplified by PCR and inserted into the BamHI and NotI sites of the vector using the primers specified in Supplementary Table 1 . Mutations into these constructs were done using whole-plasmid PCR or 2-step PCR. All constructs were verified by sequencing. The generation of stable HeLa cell lines was done using the Flp-In system (Invitrogen) and the resulting clones were kept under selection by supplementing the growth media with 200 μg ml −1 Hygromycin B and 5 μg ml −1 Blasticidin S. Antibodies The following antibodies were used for western blot, immunofluorescence or immunoprecipitation as indicated: α-tubulin 11H10 (rabbit, Cell Signaling) 1:100 IF, β-actin AC-15 (mouse, Abcam) 1:5,000 WB, APC1 A301–653A (rabbit, Bethyl) 1:500 WB, APC3 35/CDC27 (mouse, BD Biosciences) 1:250 WB, APC4 (mouse, raised against a C-terminal peptide) 5 μg IP, APC7 A302–551A (rabbit, Bethyl) 1:1,000 WB, Bub3 clone 31 (mouse, BD Transduction Laboratories) 1:500 WB, BubR1 A300–995A (rabbit, Bethyl) 1:500 WB, BubR1 A300–386A (rabbit, Bethyl) 1:200 IF, Cdc20 AR12 (mouse, Millipore) 1:200 IF/5 μg IP, Cdc20 E-7 (mouse, Santa Cruz Biotechnology) 1:500 WB, Cdc20 A301–180A (rabbit, Bethyl) 1:1,000 WB, CREST (human, Antibodies Inc.) 1:400 IF, FLAG M2 (mouse, Sigma) 1:5,000 WB, GFP clones 7.1 and 13.1 (mouse, Roche) 1:5,000 WB /1:200 IF, Mad2 from G. Kops (rabbit) 1:200 IF, Mad2 A300–301A (rabbit, Bethyl) 1:1,000 WB, p31 rabbit antibody was generated using full-length p31 as antigen and affinity purified. Full scans of western blots are presented in Supplementary Figs 5 and 6 . RNAi depletion of proteins RNAi depletion of proteins was performed for 48 h, except for p31 that was performed twice at 72 and 48 h before analysis. DMEM media was replaced with OPTIMEM media right before adding a mix containing 100 nM RNAi oligo (Sigma) and 4 μl ml −1 RNAimax (Invitrogen) diluted in OPTIMEM. The media was changed after 5 h and replaced with DMEM supplemented with 10% FBS. siRNAs used are BubR1 5′-GAUGGUGAAUUGUGGAAUA-3′; Cdc20 5′-CGGAAGACCUGCCGUUACAUU-3′; KNL1 5′-AAGAUCUGAUUAAGGAUCCACGAAA-3′; Luciferase 5′-CGUACGCGGAAUACUUCGA-3′; Mad2 5′-GGAAGAGUCGGGACCACAG-3′; p31 5′-GGCUGCUGUCAGUUUACUU-3′. Immunofluorescence analysis For immunofluorescence microscopy, cells were synchronized with 2.5 mM thymidine, 10 μM MG132 and 660 mM nocodazole as shown in Fig. 1a . Cells were pre-fixed with 4% PFA in PHEM buffer (50 mM Pipes, 25 mM Hepes, 10 mM EGTA, 8.5 mM MgSO 4 , pH 7.0) for 20 s, permeabilized in 0.5% TritonX-100 in PHEM buffer for 5 min and fixed in 4% PFA in PHEM buffer for 20 min. Coverslips were quenched with 25 mM Glycine in PBS for 20 min, blocked with 3% BSA in PBS-T (0.1% Tween in PBS) for 30 min, incubated with primary antibodies for 1 h, with Alexa Fluor goat secondary antibodies for 45 min and mounted on slides using ProLong Gold Antifade mounting media (Invitrogen). Images were acquired taking z stacks of 200 nm using a × 100/1.4NA objective on a DeltaVision Elite Microscope (GE Healthcare). Images were analysed after deconvolution using SoftWoRx (GE Healthcare). Figures were generated by maximum intensity projection of entire cells using Softworx and ImageJ. Live cell imaging Live cell analysis was performed on a Deltavision Elite system using a × 40 or × 60 objective (GE Healthcare). Cells were seeded in 8-well Ibidi dishes (Ibidi) in advance and before filming the media was changed to Leibovitz´s L-15 (Life technologies). Appropriate channels were recorded for 18 h and data analysed using Softworx (GE Healthcare). MEFs were transfected with Venus-Cdc20 proteins by electroporation using the Neon Transfection System according to the manufacturer’s instructions. 1 μM 4-OHT and 200 nM taxol were added where indicated 24 h and 2 h before filming, respectively. For experiments in Fig. 2b images were acquired on a Perkin Elmer UltraView Vox-Spinning Disk CSU-X1 using a × 60 1.4 oil objective. Immunopurification of complexes Immunoprecipitation of Venus proteins from stable HeLa cell lines was performed from cells synchronized with 2.5 mM thymidine and arrested in mitosis with either 660 mM nocodazole or 200 mM taxol. The mitotic cells were harvested by shake off, washed with ice-cold PBS and lysed for 30 min on ice in lysis buffer (150 mM NaCl, 50 mM Tris–HCl pH 7.5, 1 mM EDTA, 1% NP40, 1 mM DTT, 1 × protease inhibitor cocktail (Roche), 1 × phosphatase inhibitor cocktail (Roche)). Lysates were clarified by centrifugation at 20,000 r.c.f. at 4 °C for 15 min, and the resulting cell extracts were incubated with 20 μl of GFP-Trap A beads (ChromoTek) at 4 °C with gentle agitation for 30 min. The beads were than washed three times with ice-cold lysis buffer and the complexes eluted in 2 × SDS sample buffer. Low salt/high salt IP was performed using a different lysis buffer (50 mM NaCl, 25 mM Tris–HCl pH 7.5, 0.1% NP40, 1 mM DTT, 1 × protease inhibitor cocktail (Roche), 1 × phosphatase inhibitor cocktail (Roche)) and washing buffer (50 mM Tris–HCl pH 7.5, 1 mg ml −1 BSA, 20% glycerol, 0.5 mM DTT, 1 × protease inhibitor cocktail (Roche), 1 × phosphatase inhibitor cocktail (Roche)) supplemented with 300 mM NaCl only for the high salt condition. IP of endogenous proteins was performed using Dynabeads Protein G (Invitrogen) and 5 μg of antibodies. In vitro binding experiments with BubR1 and Cdc20 FLAG-HA-BubR1 516–715 was expressed in the E. coli BL21 Rosetta2 (DE3) R3 T1 strain by induction with 0.5 mM IPTG for 20 h at 18 °C. The bacterial pellet was resuspended in buffer L (50 mM NaP, 300 mM NaCl, 10% glycerol, 0.5 mM TCEP, protease inhibitors) and lysed using a high-pressure homogenizer at 1,000 Bar. After clarification by centrifugation (18,000 g for 30 min) the protein was purified by affinity (1 ml Ni column (GE healthcare), loaded in buffer L with 10 mM imidazole) and gel filtration chromatography (Superdex 200 PG 16/60 equilibrated with SEC buffer (50 mM NaP, 150 NaCl, 0.5 mM TCEP, 10% glycerol, pH 7.5)). Strep-His-Cdc20 and mutants thereof where expressed in HEK293 6E cell lines by transfection with 100 μg ml −1 Polyethylenimine ‘MAX’(PEI) (polysciences). After 3 days the Cdc20 proteins were affinity purified using a Strep-tag/Strep-Tactin purification system (IBA) according to manufacturer’s description. Ten micrograms of FLAG-HA-BubR1 516–715 protein was incubated with 20 μl of anti-FLAG M2 affinity gel (Sigma) in PBS for 1 h at room temperature with gentle mixing followed by three washes with washing buffer (PBS, 0.1% TritonX-100). The affinity gel was then resuspended in binding buffer (150 mM NaCl, 50 mM Tris–HCl pH 7.5, 0.3% Triton X-100, 1 × protease inhibitor cocktail (Roche), 1 × phosphatase inhibitor cocktail (Roche)) and incubated with 2, 5 or 10 μg of Strep-His-Cdc20 proteins for 1 h at room temperature with gentle mixing. After four washes with the binding buffer, the bound proteins were released from the affinity gel by addition of 2 × SDS sample buffer and incubation at 95 °C. The eluates were analysed by Coomassie staining and western blotting against BubR1 (FLAG) and Cdc20 (E7, Santa Cruz). In vitro ubiquitination assays with APC/C APC/C-Cdc20 complexes were purified from mitotic cells using an APC4 antibody. Cells were either control treated or depleted of Cdc20 by RNAi and the expression of the different Venus-Cdc20 proteins induced by doxycycline. In vitro ubiquitination assays with in vitro translated Cyclin B1 1–86 was carried out as previously described [42] . Binding experiments in HEK293 cells For experiments presented in Supplementary Fig. 3a,b HEK293T cell were transfected with Venus-BubR1 proteins and depleted of endogenous BubR1 using Lipofectamine 2000 (Invitrogen), 500 ng ml −1 plasmid and 100 nM RNAi oligo. Cells were subsequently synchronized with 2.5 mM thymidine for 24 h and treated with 200 ng ml −1 nocodazole after the thymidine release. 10 μM MG132 was added after 6 h from the thymidine release for 3 h. Cells were then harvested and washed with ice-cold PBS. Peptide binding experiments Two peptides were used for this assay: Biotin-YSVPFSIFDEFLLSEKKNKS (WT peptide) and Biotin-YSVPFSIAKKAAASEKKNKS (mut peptide) (BIOSYNTAN). Two micrograms of purified Strep-His-Cdc20 was incubated with peptide–streptavidin agarose complex (Sigma) for 1 h at room temperature. The binding buffer contains 50 mM Tris–HCl, pH=7.5, 150 mM NaCl, 0.3% TritonX-100 with protease inhibitors. After four times of washing with the binding buffer, the bound proteins were eluted by 1 × Laemmli buffer and released by incubating at 95 °C. The eluates were analysed by western blot against Cdc20 (E7, Santa Cruz). Size exclusion chromatography Cell lines were arrested in nocodazole and treated for 1 h with reversine and MG132 before harvesting. The cells were resuspended in lysis buffer (150 nM NaCl, 25 mM TRIS pH 8.0, 0.1% NP-40, 1 mM DTT, 1 × protease inhibitor cocktail (Roche) and 1 × phosphatase inhibitor cocktail (Roche)). Following lysis the extract was clarified by spinning for 10 min at 20,000 g and subsequently for 10 min at 186,000 g in a TLA-55 rotor (Beckman-Coulter). Five hundred microlitres of extract at 6 μg μl −1 was loaded on a Superose 6 10/300 GL column equilibrated with lysis buffer. Five-hundred microlitre fractions where collected and analysed. How to cite this article: Lischetti, T. et al. The internal Cdc20 binding site in BubR1 facilitates both spindle assembly checkpoint signalling and silencing. Nat. Commun. 5:5563 doi: 10.1038/ncomms6563 (2014).